NHC-catalyzed atropoenantioselective synthesis of axially chiral biaryl amino alcohols via a cooperative strategy Axially chiral biaryl amino-alcohols play a pivotal role in organic synthesis and drug discovery. However, only a very few enantioselective methods have been reported to synthesize chiral biaryl amino-alcohols. Therefore, the rapid enantioselective construction of optically active biaryl amino-alcohols still remains a formidable challenge. Here we report an N-heterocyclic carbene (NHC)-catalyzed atropoenantioselective acylation of biphenols triggered by a cooperative strategy consisting of desymmetrization followed by kinetic resolution. This protocol features broad substrate scope and good functional group tolerance, and allows for a rapid construction of axially chiral biaryl amino-alcohols in good to high yields and with excellent enantioselectivities. Furthermore, the structurally diverse axially chiral biaryl amino-alcohol derivatives provide multiple possibilities for chemists to develop catalysts or ligands for different chemical transformations. Axially chiral biaryls [1] , [2] , [3] have widely applied in many areas, including material science [4] , [5] and drug discovery [6] . In addition, chiral biaryls have often played as ligands [7] or catalysts [8] in the development of enantioselective catalytic transformations. During the past two decades, BINOL and BINAM have proven to be representative examples in this category [9] , [10] , [11] , [12] , [13] , [14] . Afterward, NOBIN (Fig. 1 ) gradually grows up to the next privileged scaffold [15] with numerous important applications, due to its perfect enantio-control and prominent bioactivity (Fig. 1 , (R)-Streptonigrin, an antitumor agent). Fig. 1 Representative molecules and synthetic protocols. a Two representative axially chiral molecules. b Asymmetric kinetic resolution of achiral biaryl amino alcohols. c Our synthetic proposal via a NHC-catalyzed atroposelective synthesis of axially chiral biaryl amino-alcohols via a cascade strategy of desymmetrization followed by kinetic resolution Full size image In sharp contrast to the asymmetric preparation of BINOL or BINAM [16] , [17] , [18] , [19] , to date, only a very few enantioselective methods have been reported to synthesize NOBIN-type biaryl amino alcohols [20] , [21] , [22] , [23] . In 1992, Kocovsky [24] and coworkers reported the asymmetric synthesis of NOBIN via oxidative of 2-naphthol with 2-naphylamine. However, the use of large excess amount of chiral auxiliary and required multistep crystallization sometimes restrict its further application. To face this issue, Tan’s group [25] uncovered a phosphoric acid-catalyzed cross-coupling of 2-naphthylamines with iminoquinones, affording chiral biaryl amino alcohols in a concise and catalytic pattern. Shortly after, optical resolution rapidly developed into the next attractive method to isolate NOBIN enantiomers by leveraging the power of diastereoisomeric chiral salt formation, but was confined to unstable reproducibility in practical [26] , [27] . Getting the NOBIN derivatives through a direct transformation from chiral raw materials (e.g., BINOL [28] or BINAM [29] ) has also become an interesting way. Regrettably, this protocol is mostly applied to construct chiral binaphthyl-type amino-alcohols. Recently, kinetic resolution is recognized as an impresive technology to produce such biaryl structures. For example, the groups of Maruoka [30] and Zhao [31] reported a phase-transfer- or N-heterocyclic carbene-catalyzed asymmetric kinetic resolution to prepare enantioenriched chiral biaryl amino alcohols, independently (Fig. 1 ). However, no more than 50% theoretical yields inevitably affect the application of this approach. Overall, rapid synthesis of axially chiral biaryl amino-alcohols in a highly atropoenantioselective fashion is still in its infancy Our group is interested in exploring carbene catalysis for the rapid assembling of axially chiral molecules. To date, we have successfully reported the N-heterocyclic carbene-catalyzed atropoenantioselective [3 + 3] annulation and kinetic resolution of anilides, affording valuable chiral α-pyrone-aryls and isoindolinones, respectively [32] , [33] . Despite aforementioned achievements, the unsolved challenges and the continuously growing demands of atropoenantiomers still drive us to develop more efficient and revolutionary protocols. We herein report a carbene-catalyzed [34] , [35] , [36] , [37] , [38] , [39] , [40] , [41] atroposelective synthesis of axially chiral biaryl amino-alcohols via a cascade strategy of desymmetrization followed by kinetic resolution [42] (Fig. 1 ). First, this approach can deliver nonclassical NOBIN derivatives (e.g., biphenyl- or phenyl-naphthyl-type amino-alcohols) in a high chemical yield. From the aspect of structural diversity, non-classical NOBIN-type derivatives will offer more possibilities for the exploration of new chiral catalysts or ligands. Second, in contrast to an independent desymmetrization or kinetic resolution method, the cooperation of desymmetrization [43] , [44] , [45] , [46] , [47] , [48] with kinetic resolution [49] , [50] , [51] , [52] , [53] has certain superiority in the control of enantioselectivity. Reaction optimization We commenced our study by using biphenols ( 1a – c ) as the model prochiral substrates, aldehyde ( 2a ) as acylation reagent [54] , [55] , [56] , [57] , [58] , [59] , [60] , [61] , [62] and DQ as oxidant [63] , [64] . 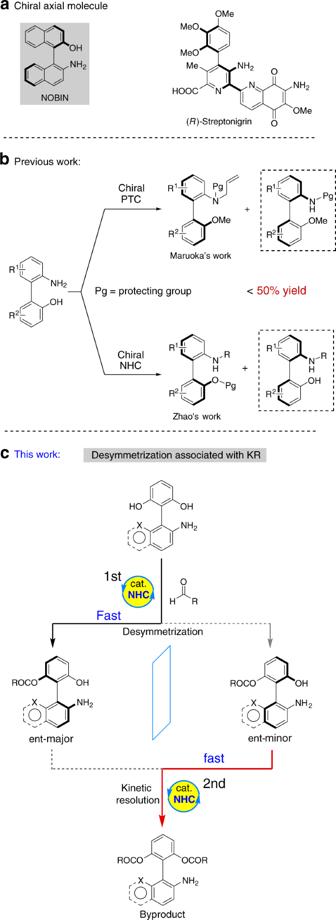Fig. 1 Representative molecules and synthetic protocols.aTwo representative axially chiral molecules.bAsymmetric kinetic resolution of achiral biaryl amino alcohols.cOur synthetic proposal via a NHC-catalyzed atroposelective synthesis of axially chiral biaryl amino-alcohols via a cascade strategy of desymmetrization followed by kinetic resolution Key results of reaction optimization are briefly summarized in Table 1 . Building upon the indanol-derived triazolium scaffold, precatalysts with N-2,4,6-(Cl) 3 C 6 H 2 [65] , or N-C 6 F 5 [66] , substituents (Table 1 , C2 and C3 ), derived from α-amino acids, were tested but exhibited low conversions and enantioselectivities (Table 1 , entries 4 and 5). Interestingly, precatalyst C1 with N-2,4,6-(Me) 3 C 6 H 2 (N-Mes) [67] substituent provided 3a in 63% with 85% ee (Table 1 , entry 1). 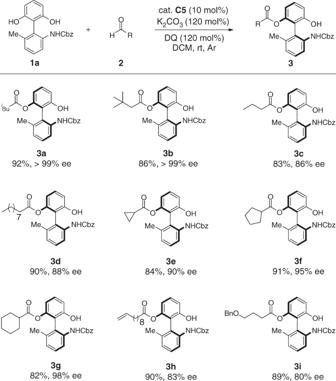Fig. 2 Scope of aldehydes. Reaction conditions: a mixture of1a(0.10 mmol),2(0.15 mmol), K2CO3(0.12 mmol), and DQ (0.12 mmol) in CH2Cl2(1.0 mL) was stirred at room temperature under N2for 12–24 h If substrate 1b or 1c replaced 1a (R = NO 2 or NH 2 ; More information about changing R groups, see Supplementary Table 2 ), low ee and yield were observed (Table 1 , entries 2 and 3). To our delight, further improved enantioselectivities were achieved with the N-2,4,6-( i Pr) 3 C 6 H 2 substituted catalyst C4 or C5 [68] (Table 1 , entries 6 and 7). Notably, the triazolium catalyst C5 , which bears a strong electron-withdrawing group (NO 2 ) at the remote aryl position, afforded 95% ee and 80% yield (Table 1 , entry 7). We then chose catalyst C5 , substrate 1a and 2a for further optimization. After extensive screening of solvents, bases and catalyst loading, an ideal result was obtained by using 10 mol% of C5 as catalyst, DCM as the solvent, and K 2 CO 3 as the base (Table 1 , entry 15). Meanwhile, nuclear magnetic resonance (NMR) spectrum confirmed that the main byproduct of this reaction was a bisadduct in which two hydroxyl groups were both acylated (see Supplementary Note 4). Table 1 Optimization of the reaction conditions a Full size table Substrate scope Having the optimal condition in hand, we turned our attention to the generality of aldehydes. As indicated in Fig. 2 , a diverse set of aliphatic aldehydes underwent acylating reactions, affording their corresponding products in high yields with high to excellent ee values (Figs. 2 and 3b–i ). Unambiguously, the steric effect of aldehydes has identified to be a critical factor for achieving high enantioselectivity. Aliphatic aldehydes bearing a steric bulky chain afforded a higher ee value (Figs. 2 and 3a, b, f, g ). When aromatic aldehydes were used as substrates, reactions are generally messy, probably caused by the competitive benzoin reaction. Fig. 2 Scope of aldehydes. Reaction conditions: a mixture of 1a (0.10 mmol), 2 (0.15 mmol), K 2 CO 3 (0.12 mmol), and DQ (0.12 mmol) in CH 2 Cl 2 (1.0 mL) was stirred at room temperature under N 2 for 12–24 h Full size image Fig. 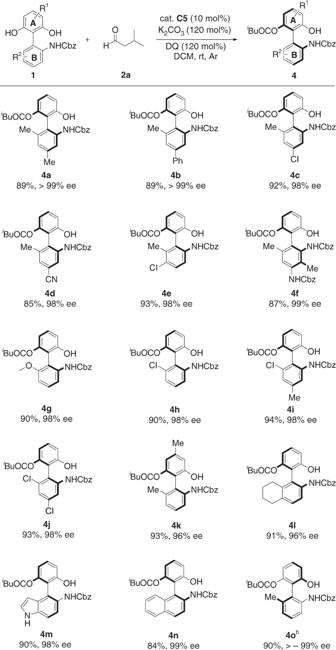Fig. 3 Scope of biaryl biphenols. Reaction conditions: a mixture of4a–4o(0.10 mmol),2a(0.15 mmol), K2CO3(0.12 mmol), and DQ (0.12 mmol) in CH2Cl2(1.0 mL) was stirred at room temperature under N2for 12–24 h.bent-cat.C5was used 3 Scope of biaryl biphenols. Reaction conditions: a mixture of 4a – 4o (0.10 mmol), 2a (0.15 mmol), K 2 CO 3 (0.12 mmol), and DQ (0.12 mmol) in CH 2 Cl 2 (1.0 mL) was stirred at room temperature under N 2 for 12–24 h. b ent-cat. C5 was used Full size image Encouraged by success with aliphatic aldehydes, we then planed to investigate the reactivity of biaryl-type biphenol substrates. N-Cbz protected compounds 4a–j having electron-donating groups (Me, MeO) and/or electron-withdrawing groups (Cl, CN) on the lower ring (Fig. 3 , phenyl ring B) generated the coresponding products in high yields (85 – 94%) with excellent enantioselectivities (96– >99% ee). Cyclohexane ring fused biphenyl substrate also performed well as expected (Fig. 3 , 4l , 91% yield and 96% ee). Pleasingly, the indole-based biaryl substrate also proceeded smoothly to afford product 4m with a promising ee value. Gratifyingly, the phenyl-naphthalenyl-type biaryl substrate was also tolerated to deliver the anticipated structure 4n with excellent enantioselectivity (Fig. 3 , 99% ee). Incidentally, enantiomeric products can be achieved entirely through the enantiomer catalyst and similar reaction conditions (Fig. 3 , 4o ). Mechanistic studies To verify the mechanism, two control experiments were conducted. As indicated in Fig. 1a , 4 ), ent- 3a was obtained in 49% yield with 93% ee in the presence of DQ (0.6 equiv). On the basis of these data, we can conclude that desymmetrization is a key contributor for enantio-control ( V fast / V slow = 28:1) [69] . Meanwhile, we also wonder whether the second acylation is a kinetic resolution process, eventually resulting in an improved enantioselectivity. To approve this hypothesis, the control experiment of (±)- 3a with 2a was designed and carried out, generating ent- 3a in 47% yield with 76% ee (Fig. 1a , 4 ). This experiment result suggests that the conversion of 1a to major enantiomer 3a is much faster than the process between 1a and minor enantiomer ( V fast / V slow = 5:1) [69] . Fig. 4 Postulated mechanistic pathways. a The control experiments (Eqs. 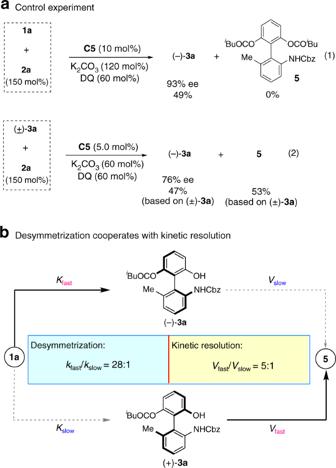Fig. 4 Postulated mechanistic pathways.aThe control experiments (Eqs. (1) and (2)) show that the desymmetrization process is the main contributor to the observed ee of the product and the second acylation is a effective KR process that could improve the ee of (−)-3a.bThe postulated mechanistic pathway to generate product (−)-3a (1) and (2)) show that the desymmetrization process is the main contributor to the observed ee of the product and the second acylation is a effective KR process that could improve the ee of (−)- 3a . b The postulated mechanistic pathway to generate product (−)- 3a Full size image Synthetic transformations and applications We anticipated that the biaryl amino-alcohol 7 (Fig. 5 ), prepared from 4n via a N-Cbz protected intermediate 6 , could be directly utilized as a chiral catalyst in asymmetric alkylation reaction. As highlighted in Fig. 6 , compound 7 successfully catalyzed the asymmetric alkylation of Ni-complex 8 with alkyl bromide 9 – 11 to generate complex 12 – 14 with promising er values. After a subsequent deprotection, 12 – 14 could efficiently transfer to valuable chiral α-amino acids [70] . To further expand synthetic utility, we conducted a Ru-catalyzed asymmetric reduction of ketone 18 by using chiral biaryl amino-alcohol derivatives 15 – 17 as ligands (for preparation of 15 – 17 , see Supplementary Note 5 ). As indicated in Fig. 6 , ligands 15 – 17 led to the corresponding product 19 in suggestable er values. In addition, a gram-scale synthesis (3.4 mmol) carried out under standard conditions afforded optically pure 3a in a pleasant result (Fig. 7 , 89% yield, 99% ee). The absolute configuration of derivative 6 was determined by X-ray single crystal analysis (See Supplementary Fig. 1 ), and other structures were assigned by analogy. Fig. 5 Synthetic transformations. Reaction conditions: (1) 4n , TMSCHN 2 , CHCl 3 :MeOH/5:1, r.t., 24 h. (2) NaOMe, MeOH, r.t., 1.0 h. (3) Pd/C, H 2 , MeOH, r.t., 3.0 h Full size image Fig. 6 Synthetic applications. a Use of 7 as a chiral catalyst. b Utility of 15 – 17 as chiral ligands Full size image Fig. 7 Gram-scale synthesis. Reaction conditions: a mixture of 1a (3.4 mmol, 1.19 g), 2a (5.1 mmol, 0.55 mL), in CH 2 Cl 2 (34.0 mL) was stirred at room temperature for 15 h Full size image In conclusion, we have developed an atropoenantioselective NHC-catalyzed acylation for the preparation of axially chiral biaryl amino-alcohols. The cascade strategy of desymmetrization followed by kinetic resolution could efficiently deliver axially chiral biaryl amino-alcohols with high to excellent ee values (up to >99% ee). Further studies on the exploration of other substrates and applications are ongoing projects in our laboratory. Synthesis of racemic ¾ In a glovebox, a flame-dried Schlenk reaction tube equipped with a magnetic stir bar, were added racemic NHC precatalyst C13 (0.01 mmol,), K 2 CO 3 (16.6 mg, 0.12 mmol), oxidant DQ (49.0 mg, 0.12 mmol), 1 (0.10 mmol), 2 (0.15 mmol), and freshly distilled CH 2 Cl 2 (1.0 mL). The reaction mixture was stirred at room temperature for 12 h. The mixture was then filtered through a pad of Celite washed with CH 2 Cl 2 . After solvent was evaporated, the residue was purified by flash column chromatography to afford the racemic product 3/4 . Synthesis of ¾ In a glovebox, a flame-dried Schlenk reaction tube equipped with a magnetic stir bar, were added NHC precatalyst C5 (0.01 mmol,), K 2 CO 3 (16.6 mg, 0.12 mmol), oxidant DQ (49.0 mg, 0.12 mmol), 1 (0.10 mmol), 2 (0.15 mmol), and freshly distilled CH 2 Cl 2 (1.0 mL). The reaction mixture was stirred at room temperature until the starting material 1 was completely consumed (12–24 h). 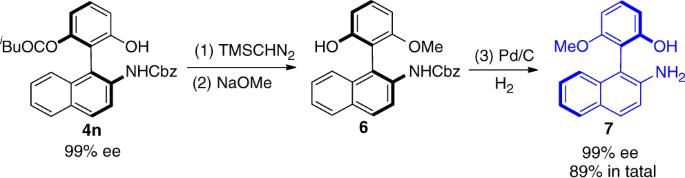Fig. 5 Synthetic transformations. Reaction conditions: (1)4n, TMSCHN2, CHCl3:MeOH/5:1, r.t., 24 h. (2) NaOMe, MeOH, r.t., 1.0 h. (3) Pd/C, H2, MeOH, r.t., 3.0 h The mixture was then filtered through a pad of Celite washed with CH 2 Cl 2 . 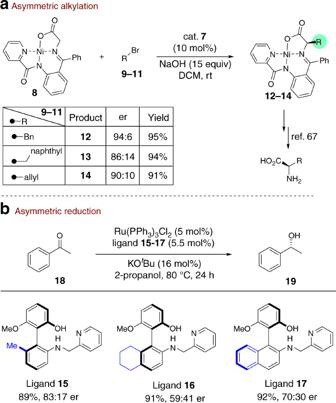Fig. 6 Synthetic applications.aUse of7as a chiral catalyst.bUtility of15–17as chiral ligands 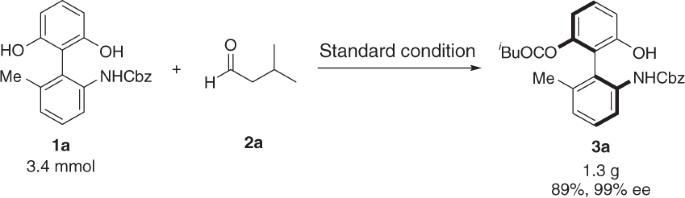Fig. 7 Gram-scale synthesis. Reaction conditions: a mixture of1a(3.4 mmol, 1.19 g),2a(5.1 mmol, 0.55 mL), in CH2Cl2(34.0 mL) was stirred at room temperature for 15 h After solvent was evaporated, the residue was purified by flash column chromatography to afford the desired product 3/4 .